A role for T-bet-mediated tumour immune surveillance in anti-IL-17A treatment of lung cancer Lung cancer is the leading cause of cancer deaths worldwide. The cytokine interleukin-17A supports tumour vascularization and growth, however, its role in lung cancer is unknown. Here we show, in the lungs of patients with lung adenocarcinoma, an increase in interleukin-17A that is inversely correlated with the expression of T-bet and correlated with the T regulatory cell transcription factor Foxp3. Local targeting of interleukin-17A in experimental lung adenocarcinoma results in a reduction in tumour load, local expansion of interferon-γ-producing CD4 + T cells and a reduction in lung CD4 + CD25 + Foxp3 + regulatory T cells. T-bet (−/−) mice have a significantly higher tumour load compared with wild-type mice. This is associated with the local upregulation of interleukin-23 and induction of interleukin-17A/interleukin-17R-expressing T cells infiltrating the tumour. Local anti-interleukin-17A antibody treatment partially improves the survival of T-bet (−/−) mice. These results suggest that local anti-interleukin-17A antibody therapy could be considered for the treatment of lung tumours. Lung cancer is the leading cause of cancer deaths worldwide and lung adenocarcinoma is one of the predominant forms [1] , [2] , [3] . Given the well-established immunosuppressive properties of the tumour environment, strategies to reverse these events by stimulating host immune responses are of potential relevance. Although the role of Th 17 cells in autoimmunity has been intensively studied [4] , [5] , their role in tumour development remains largely unknown. Previous reports have shown that both cutaneous T-cell lymphomas [6] and ovarian carcinomas [7] spontaneously secrete interleukin (IL)-17A and in a considerable proportion of ovarian tumours IL-17A expression correlates with increased vascularity. However, no report exists concerning a possible angiogenic role for IL-17A in non-small cell lung cancer (NSCLC) [8] , [9] , [10] . NSCLC cells have been reported to produce many angiogenic factors, including CXCL8/IL-8 (refs 11 , 12 ), which are critically involved in the pathogenesis of NSCLC [13] . It has been reported that inhibition of CXCL8 suppressed the growth of NSCLC in immunodeficient mice [14] . Conversely, tumour-derived CXCL10/interferon (IFN)-inducible protein-10 has been identified as an important endogenous angiostatic factor in NSCLC [15] . As IL-17A induces CXCL8 production and CXCL8 is involved in the angiogenic activity of NSCLC [16] , we asked whether IL-17A might be increased and may contribute to the development of lung adenocarcinoma. Thus, we analysed the role of Th 17 cells in a murine model of lung adenocarcinoma and human tumours. We identified T-bet as an antagonist of IL-17A/IL-17R expression that inhibits T regulatory cell development in lung tumours. In vivo targeting of IL-17A abrogated tumour growth in the presence of T-bet by inhibiting CD4 + CD25 + Foxp3 + T regulatory cells and inducing IFN-γ and tumour necrosis factor-α (TNFα) production by CD4+ T cells. In the absence of T-bet, anti-IL-17A antibody therapy inhibited IL-17R expression on CD4 + and induced IFN-γ in lung CD8+ T cells and improved survival in a murine model of lung cancer. Taken together, anti-IL-17A antibody therapy emerges as a promising avenue in the treatment of lung cancer. Expression of ROR transcription factors and IL-17A in adenocarcinoma To address the role of Th 17 immune responses in tumours, we used quantitative PCR to measure the expression of Th 17 cell [17] lineage-specific transcription factors RORα4 and RORC2 (human homologue of mouse RORγt), as well as IL-17A, in lung samples derived from patients with lung adenocarcinoma or healthy control tissue. 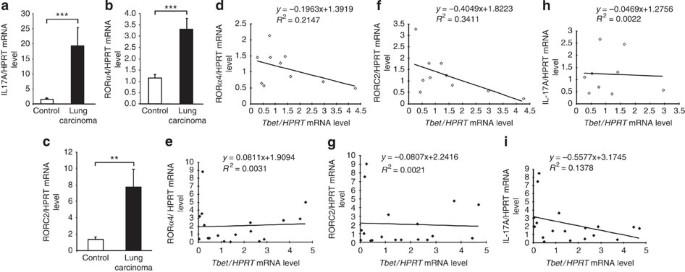Figure 1: Increased expression of Th17 markers in lungs of adenocarcinoma patients. RNA from tumour tissue biopsy samples of patients suffering from lung adenocarcinoma and healthy control lung tissues was extracted and analysed by qPCR. mRNA levels of (a) IL-17A (Ncontrol=9;Nlung carcinoma=25), (b) RORα4 (Ncontrol=10;Nlung carcinoma=25) and (c) RORC2 (Ncontrol=10;Nlung carcinoma=25) are shown. Data are reported as mean values±s.e.m. Student's two-tailedt-test was used. **P,0.01; ***P,0.001. (d) Correlation between T-bet and RORα4 mRNA expression in control lung tissue (open symbols) (N=10) compared with adenocarcinoma-bearing lung tissue (filled symbols) (e;N=18), between T-bet and RORC2 in healthy samples (f;N=10) and carcinoma samples (g;N=18) and between T-bet and IL-17A in healthy controls (h;N=9) and adenocarcinoma tissue (i;N=18). Values of individual patients are shown. The correlations are indicated. The clinical characteristics of the subjects are reported in Table 1 . Table 1 Clinical characteristics of the patients used in this human study. Full size table We found that patients with lung adenocarcinoma had a significant increase in IL-17A, RORα4 and RORC2 mRNA expression in the lung compared with control subjects ( Fig. 1a–c , respectively). Noteworthy was the tenfold increase in IL-17A mRNA in tumour samples suggesting a local induction of Th 17 responses at the transcriptional level. Figure 1: Increased expression of Th17 markers in lungs of adenocarcinoma patients. RNA from tumour tissue biopsy samples of patients suffering from lung adenocarcinoma and healthy control lung tissues was extracted and analysed by qPCR. mRNA levels of ( a ) IL-17A ( N control =9; N lung carcinoma =25), ( b ) RORα4 ( N control =10; N lung carcinoma =25) and ( c ) RORC2 ( N control =10; N lung carcinoma =25) are shown. Data are reported as mean values±s.e.m. Student's two-tailed t -test was used. ** P ,0.01; *** P ,0.001. ( d ) Correlation between T-bet and RORα4 mRNA expression in control lung tissue (open symbols) ( N =10) compared with adenocarcinoma-bearing lung tissue (filled symbols) ( e ; N =18), between T-bet and RORC2 in healthy samples ( f ; N =10) and carcinoma samples ( g ; N =18) and between T-bet and IL-17A in healthy controls ( h ; N =9) and adenocarcinoma tissue ( i ; N =18). Values of individual patients are shown. The correlations are indicated. Full size image As previous studies had identified T-bet as a negative regulator of IL-17A in the lung [18] , we then investigated whether the increase of IL-17A, RORC2 and RORα4 in lung carcinoma was secondary to a downregulation of T-bet in the lung tissue. Accordingly, we examined correlations between T-bet, IL-17A, RORα4 and RORC2 expression in tumour samples and healthy control tissues. RORα4 and RORC2 had higher values when T-bet expression was low in normal control lung tissues ( Fig. 1d,f , respectively). These data indicated a reciprocal inhibitory role of T-bet on RORC2 and RORα4 in normal tissue. However, in tumour tissues, these inverse correlations were lost, indicating that RORα4 and RORC2 in lung tumour expanded independently from T-bet ( Fig. 1e,g , respectively). We next analysed the correlation between IL-17A and T-bet and found that in control lung tissues T-bet does not decrease when IL-17A is increased ( Fig. 1h ). However, we found an inverse correlation between T-bet and IL-17A expression in tumour samples indicating that low values of T-bet occur with high IL-17A expression in human lung tumours ( Fig. 1i ). Increased Foxp3 mRNA transcription in lung adenocarcinoma tissue To understand the potential relationship between Th 17 development and the suppressor regulatory Foxp3 + CD4 + T (T reg ) cells in tumour tissues, we next analysed the expression of the signature transcription factor of T reg cells, Foxp3, in the same human lung tissues where we analysed IL-17A levels. Foxp3 mRNA expression was significantly increased in lung adenocarcinoma samples compared with control samples ( Fig. 2a ). Furthermore, a strong positive correlation was found between Foxp3 and RORC2 ( Fig. 2b,c ) and between Foxp3 and IL-17A mRNA expression ( Fig. 2d,e ) in lung adenocarcinoma samples compared with control samples. This finding suggests a synergy between Th 17 and T reg cells in lung adenocarcinoma in the presence of low T-bet levels. 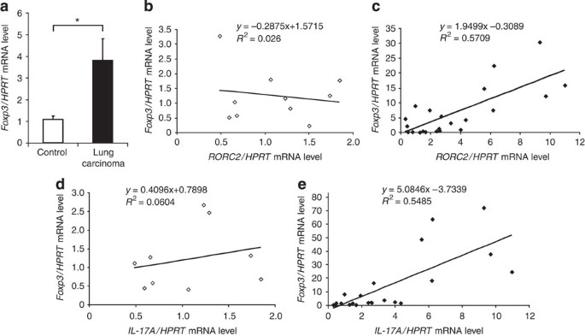Figure 2: Increased Foxp3 expression in lungs of adenocarcinoma patients correlates with IL-17A and RORC2. Lung mRNA from patients with adenocarcinoma (filled symbols) and control lung tissues (open symbols) was extracted and analysed by quantitative PCR. (a) mRNA expression levels of Foxp3 in human control and adenocarcinoma-bearing lung tissue biopsy samples (Ncontrol=10;Nlung carcinoma=22). Data are presented as mean values±s.e.m. Student's two-tailedt-test was used. *P,0.05. (b) Correlation between Foxp3 and RORC2 mRNA expression in control lung tissue (N=10) and (c) adenocarcinoma-bearing tissue (N=22), correlation between Foxp3 and IL-17A mRNA expression in healthy controls (d;N=9) and carcinoma tissue (e;N=20). Values of individual patients are shown. The correlations are indicated. Figure 2: Increased Foxp3 expression in lungs of adenocarcinoma patients correlates with IL-17A and RORC2. Lung mRNA from patients with adenocarcinoma (filled symbols) and control lung tissues (open symbols) was extracted and analysed by quantitative PCR. ( a ) mRNA expression levels of Foxp3 in human control and adenocarcinoma-bearing lung tissue biopsy samples ( N control =10; N lung carcinoma =22). Data are presented as mean values±s.e.m. Student's two-tailed t -test was used. * P ,0.05. ( b ) Correlation between Foxp3 and RORC2 mRNA expression in control lung tissue ( N =10) and ( c ) adenocarcinoma-bearing tissue ( N =22), correlation between Foxp3 and IL-17A mRNA expression in healthy controls ( d ; N =9) and carcinoma tissue ( e ; N =20). Values of individual patients are shown. The correlations are indicated. Full size image T-bet protected mice from lung tumour development To explore the role of T-bet and IL-17A in vivo , we injected L1C2 adenocarcinoma cells into T-bet (−/−) and wild-type mice and found that tumour growth was markedly affected in the absence of T-bet [19] . In an initial series of studies, 14 days after tumour cell injection, 50% of the lung surface was occupied by a tumour in T-bet (−/−) mice, whereas wild-type controls had less than 10% of lung surface occupied by tumour tissue under the same conditions ( Fig. 3a ). These data extend previous studies on lung metastasis in experimental melanoma in T-bet-deficient mice [20] , [21] , demonstrating that T-bet protects against lung tumour growth. 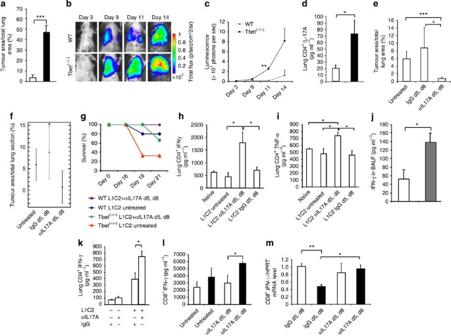Figure 3: Anti-IL-17A antibody treatment reduced tumour growth and induced IFNγ production in tumour-infiltrating CD4+T cells. (a) Histological analysis of lungs from wild-type (open column) and T-bet(−/−)(filled column) mice injected with L1C2 tumour cells (N=3–6 per group; 5 replicates). (b) Wt and T-bet(−/−)mice were injected with LL/2-luc-M38 cells and luciferase activity was measured (N=2–4). (c) Luminescence quantification of panelb. (d) IL-17A protein levels in supernatants of wt (open column) and T-bet(−/−)(filled column) L1C2 tumour-infiltrating lung CD4+T cells cultured 24 h with αCD3/αCD28 antibodies (N=3–6 per group). (e) Quantification of tumour area in lung sections of wt L1C2-bearing mice treated on days 5 and 8 with αIL17A or IgG antibodies (mean of six experiments; 8–21 per group). (f) Plot of analysis of the variance of data ine. (g) Survival of wt and T-bet(−/−)mice bearing L1C2 tumour treated with αIL-17A antibody (N=2–3 per group). (h,i) IFN-γ (h) and TNFα (i) levels released after 24 h by lung CD4+T cells isolated from naive untreated or L1C2-tumour-bearing wt mice treated with αIL-17A or IgG antibody (N=2–3 per group; representative of 2). (j) IFN-γ levels in broncho-alveolar lavage fluid (BALF) of wt (open column) and IL-17A(−/−)(grey column) mice injected with LLC1 cells (N=3–4 per group). (k) Wt mice were injected with L1C2 cells and after 6 days isolated lung CD4+T cells were cultured for 3 days with αCD3/αCD28 antibodies, IL-2 and αIL-17A or IgG. Supernatants were analysed for IFN-γ (N=3 per group). (l) IFN-γ levels of lung CD8+T cells isolated from wt (open columns) and T-bet(−/−)(filled columns) L1C2-tumour-bearing mice and cultured 24 h with αCD3/αCD28 antibodies (N=2–3 per group). (m) IFN-γ mRNA expression of L1C2-bearing wt (open columns) and T-bet(−/−)(filled columns) mice treated with IgG or αIL-17A antibody (pool of 3 experiments). For the antibody and IgG treatment 3 μg per day per mice was used. d=day. Data are shown as mean values±s.e.m. Student's two-tailedt-test was used for panelsa–eandg–m. *P,0.05; **P,0.01; ***P,0.001. Figure 3: Anti-IL-17A antibody treatment reduced tumour growth and induced IFNγ production in tumour-infiltrating CD4 + T cells. ( a ) Histological analysis of lungs from wild-type (open column) and T-bet (−/−) (filled column) mice injected with L1C2 tumour cells ( N =3–6 per group; 5 replicates). ( b ) Wt and T-bet (−/−) mice were injected with LL/2-luc-M38 cells and luciferase activity was measured ( N =2–4). ( c ) Luminescence quantification of panel b . ( d ) IL-17A protein levels in supernatants of wt (open column) and T-bet (−/−) (filled column) L1C2 tumour-infiltrating lung CD4 + T cells cultured 24 h with αCD3/αCD28 antibodies ( N =3–6 per group). ( e ) Quantification of tumour area in lung sections of wt L1C2-bearing mice treated on days 5 and 8 with αIL17A or IgG antibodies (mean of six experiments; 8–21 per group). ( f ) Plot of analysis of the variance of data in e . ( g ) Survival of wt and T-bet (−/−) mice bearing L1C2 tumour treated with αIL-17A antibody ( N =2–3 per group). ( h , i ) IFN-γ ( h ) and TNFα ( i ) levels released after 24 h by lung CD4 + T cells isolated from naive untreated or L1C2-tumour-bearing wt mice treated with αIL-17A or IgG antibody ( N =2–3 per group; representative of 2). ( j ) IFN-γ levels in broncho-alveolar lavage fluid (BALF) of wt (open column) and IL-17A (−/−) (grey column) mice injected with LLC1 cells ( N =3–4 per group). ( k ) Wt mice were injected with L1C2 cells and after 6 days isolated lung CD4 + T cells were cultured for 3 days with αCD3/αCD28 antibodies, IL-2 and αIL-17A or IgG. Supernatants were analysed for IFN-γ ( N =3 per group). ( l ) IFN-γ levels of lung CD8 + T cells isolated from wt (open columns) and T-bet (−/−) (filled columns) L1C2-tumour-bearing mice and cultured 24 h with αCD3/αCD28 antibodies ( N =2–3 per group). ( m ) IFN-γ mRNA expression of L1C2-bearing wt (open columns) and T-bet (−/−) (filled columns) mice treated with IgG or αIL-17A antibody (pool of 3 experiments). For the antibody and IgG treatment 3 μg per day per mice was used. d=day. Data are shown as mean values±s.e.m. Student's two-tailed t -test was used for panels a – e and g – m . * P ,0.05; ** P ,0.01; *** P ,0.001. Full size image In an additional approach [22] , we performed in vivo imaging of tumour cells to visualize, monitor and quantify the tumour load in the lungs of T-bet (−/−) and wild-type mice. We used a similar model of lung carcinoma where lung tumours were induced by the intravenous injection of the luciferase-expressing lung carcinoma cell line LL/2-luc-M38. In these studies, we confirmed an increased tumour load in the lung of T-bet (−/−) mice at different time points compared with control wild-type mice ( Fig. 3b,c ). Taken together, these data demonstrated that T-bet protects from tumour development in experimental lung adenocarcinoma. T-bet suppressed IL-17A production in CD4 + T cells in lung tumours Because T-bet inversely correlated with IL-17A in human lung adenocarcinoma, we next analysed IL-17A release in the supernatants of lung CD4 + T cells isolated from wild-type and T-bet-deficient mice-harbouring tumours. We found a significant upregulation of IL-17A production in CD4 + T cells isolated from T-bet (−/−) mice bearing tumours compared with those isolated from wild-type littermates ( Fig. 3d ). These results indicated that the Th 17 pathway is expanded in the absence of T-bet in this lung adenocarcinoma model. Local targeting of IL-17A suppressed lung tumour growth To investigate whether Th 17 cells are involved in the pathogenesis of lung adenocarcinoma, we treated wild-type mice with lung adenocarcinoma intranasally with a neutralizing anti-IL-17A antibody and analysed tumour development ( Fig. 3e ). We observed a statistically significant reduction of tumour growth after intranasal (i.n.) treatment of lung tumours with anti-IL-17A antibodies as compared with untreated and IgG-treated mice ( Fig. 3f ). Anti-IL-17A antibody treatment partially rescued T-bet (−/−) mice We then analysed the survival of wild-type and T-bet-deficient mice after in vivo i.n. administration of anti-IL-17A antibodies. We found that T-bet (−/−) mice have very low survival rates compared with wild-type littermates bearing tumour. At day 19 after tumour cell injection, anti-IL-17A antibody treatment rescued all wild-type and T-bet-deficient mice bearing tumours. Two days later, however, all wild-type mice treated with anti-IL-17 antibody survived, whereas only 30% of the T-bet-deficient mice died. We thus concluded that T-bet contributes to the survival achieved by anti-IL-17A antibody treatment in this model of experimental lung cancer ( Fig. 3g ). IL-17A antibody induced IFNγ production by CD4 + T cells in tumours We then asked whether blockade of IL-17A function would favour Th 1 cytokine production. We detected a statistically significant increase in both IFN-γ ( Fig. 3h ) and TNFα ( Fig. 3i ) protein levels in the supernatants of lung CD4 + T cells isolated from in vivo anti-IL-17A antibody-treated mice bearing tumours, when compared with untreated and IgG-treated mice. In addition, in a similar model of lung carcinoma, where the Lewis carcinoma cell line (LLC1) was injected [23] , targeted deletion of IL-17A led to induction of IFN-γ levels in the airways ( Fig. 3j ) confirming a negative regulatory role of IL-17A on IFN-γ production in this lung tumour model. We next isolated lung CD4 + T cells both from untreated and tumour-bearing mice and treated these cells either with anti-IL-17A or immunoglobulin G (IgG) antibodies for 3 days in vitro ( Fig. 3k ). Interestingly, only CD4 + T cells isolated from the lungs of mice with tumours, that were treated in vitro with anti-IL-17A antibody, produced high levels of IFN-γ ( Fig. 3k ). We thus demonstrate that tumour-infiltrating CD4 + T cells are direct target of anti-IL-17A therapy and this treatment favoured the production of IFN-γ by lung CD4 + T cells in experimental lung cancer. IFN-γ production in lung CD8 + T-bet (−/−) tumour T cells We next isolated lung CD8 + T cells from wild-type and T-bet-deficient mice bearing tumours treated with anti-IL-17A antibodies. We found that lung CD8 + T cells from T-bet-deficient mice produced more IFN-γ protein compared with those isolated from wild-type littermates after anti-IL-17A antibody treatment in this lung tumour model ( Fig. 3l ). Moreover, at the RNA level we could show that anti IL-17A treatment induced IFN-γ production in lung CD8 + T cells only in T-bet-deficient mice ( Fig. 3m ). These results indicated a T-bet-independent regulation of IFN-γ production in CD8 + T cells. Anti-IL-17A antibody reduced IL-6 levels in lung tumours We next analysed the influence of IL-17A on lung cells and tumour cells that were used to induce lung tumours (L1C2 and LLC1). In initial studies we focused on IL-6, a cytokine produced by Th 17 cells, which inhibits T regulatory cells and induces Th 17 cells. 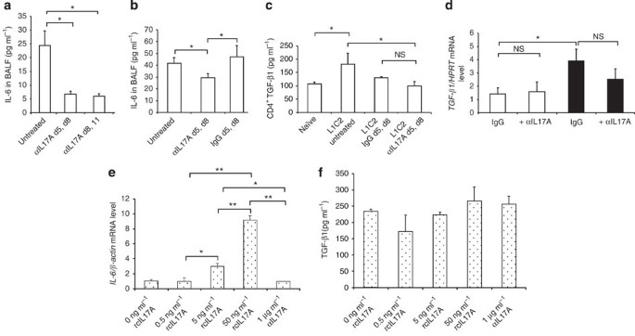Figure 4: Lung tumour cells provide an IL-6-enriched cytokine milieu to maintain Th17 cells in response to IL-17A. (a) Balb/cJ wt mice bearing L1C2 lung carcinoma were treated with αIL-17A antibodies on days 5 and 8 or on days 8 and 11 (3 μg/day) or left untreated after tumour cell injection. On day 21 IL-6 protein levels were measured in the broncho-alveolar lavage fluid (BALF) (N=3–6 per group; representative of 2 experiments). (b) IL-6 protein levels in the BALF of wt mice analysed 21 days after injection of the tumour cell line L1C2 andin vivotreated on days 5 and 8 either with IgG or αIL-17A antibodies or untreated controls (N=3–6 per group, representative of 2 experiments). (c) CD4+T cells were isolated from wt naive untreated or L1C2-tumour-bearing mice treated with IgG or αIL17A antibodies (3 μg per day) on days 5 and 8 after tumour cell injection andin vitrostimulated for 24 h with αCD3/αCD28 antibodies (N=3–6 per group). (d) Total lung TGF-β1 mRNA expression of wild-type (open columns) and T-bet(−/−)(filled columns) mice bearing tumours. Mice were treated with IgG or αIL-17A antibodies (3 μg per day) on days 5 and 8 after tumour cell injection (N=2–5 per group). (e) L1C2 cells were cultured for 48 h with different doses of recombinant IL-17A or αIL-17A antibodies, as indicated. Gene expression analysis of IL-6 mRNA was performed by qPCR (representative of two independent experiments). (f) TGF-β1protein levels of L1C2 cells cultured for 48 h with indicated amounts of rcIL17A or αIL17A antibodies (representative of two independent experiments). Data are shown as mean values±s.e.m. Student's two-tailedt-test was used. *P,0.05; **P,0.01. As shown in Figure 4a,b , in vivo treatment with anti-IL-17A antibodies significantly reduced IL-6 production in the airways (broncho-alveolar lavage fluid). Furthermore, transforming growth factor (TGF)-β 1 was increased in the supernatants of CD4 + T cells isolated from the lungs of wild-type mice bearing tumours. In addition, decreased levels of this cytokine were noted in the supernatants of lung CD4 + T cells isolated from anti-IL-17A antibody but not from IgG control-treated mice, compared with untreated tumour-bearing mice ( Fig. 4c ). Figure 4: Lung tumour cells provide an IL-6-enriched cytokine milieu to maintain Th17 cells in response to IL-17A. ( a ) Balb/cJ wt mice bearing L1C2 lung carcinoma were treated with αIL-17A antibodies on days 5 and 8 or on days 8 and 11 (3 μg/day) or left untreated after tumour cell injection. On day 21 IL-6 protein levels were measured in the broncho-alveolar lavage fluid (BALF) ( N =3–6 per group; representative of 2 experiments). ( b ) IL-6 protein levels in the BALF of wt mice analysed 21 days after injection of the tumour cell line L1C2 and in vivo treated on days 5 and 8 either with IgG or αIL-17A antibodies or untreated controls ( N =3–6 per group, representative of 2 experiments). ( c ) CD4 + T cells were isolated from wt naive untreated or L1C2-tumour-bearing mice treated with IgG or αIL17A antibodies (3 μg per day) on days 5 and 8 after tumour cell injection and in vitro stimulated for 24 h with αCD3/αCD28 antibodies ( N =3–6 per group). ( d ) Total lung TGF-β1 mRNA expression of wild-type (open columns) and T-bet (−/−) (filled columns) mice bearing tumours. Mice were treated with IgG or αIL-17A antibodies (3 μg per day) on days 5 and 8 after tumour cell injection ( N =2–5 per group). ( e ) L1C2 cells were cultured for 48 h with different doses of recombinant IL-17A or αIL-17A antibodies, as indicated. Gene expression analysis of IL-6 mRNA was performed by qPCR (representative of two independent experiments). ( f ) TGF-β 1 protein levels of L1C2 cells cultured for 48 h with indicated amounts of rcIL17A or αIL17A antibodies (representative of two independent experiments). Data are shown as mean values±s.e.m. Student's two-tailed t -test was used. * P ,0.05; ** P ,0.01. Full size image Although no statistical difference in TGF-β release was seen between the anti IL-17A antibody and IgG control-treated mice ( Fig. 4c ), TGF-β mRNA expression was upregulated in the lung of T-bet-deficient mice compared with wild-type littermates bearing tumour ( Fig. 4d ). Moreover, anti-IL-17A antibody treatment did not reduce TGF-β mRNA levels in lung tumour tissue isolated from both wild-type and T-bet-deficient mice ( Fig. 4d ). Although Th17 cells have been shown to promote cytotoxic T cell responses in a model of melanoma metastasis [24] , IL-17A has been found to favour tumour development in other models [25] , [26] , [27] . In fact, it has been previously reported that IL-17A boosts tumour development by inducing a tumour-promoting microenvironment [25] and that targeted deletion of IL-17A suppresses intestinal tumourigenesis [26] . Consistent with a pro-tumour function of IL-17A, it has also been reported that IL-17A expression is regulated by STAT3, a proto-oncogene activated by IL-6 in tumour and tumour stromal cells, promoting tumour cell survival, proliferation and angiogenesis [28] , [29] . Moreover, IL-6 has been shown to be produced by tumour cell lines upon stimulation with IL-17A (ref. 27 ). Consistently, we found a significant upregulation of IL-6 mRNA expression in the tumour cell line L1C2 after stimulation with increasing doses of IL-17A ( Fig. 4e ). In contrast, protein analysis of TGF-β in the tumour cell supernatants showed a spontaneous release of TGF-β protein but these baseline values were not significantly changed by application of IL-17A ( Fig. 4f ). Taken together, these data suggested the presence of the Th17 inducing cytokines IL-6 and TGF-β in the lung of L1C2-tumour-bearing mice by T cell- and tumour cell-dependent sources. T-bet-dependent proliferation of lung CD4 + T cells in tumours To further explore a potential relationship between Th 17 and T reg cells in lung cancer in the presence and absence of T-bet, we analysed the influence of IL-17A on lung CD4 + T cell proliferation in the tumour model. The potential relevance of this point is highlighted by the observation that Foxp3-expressing T regulatory cells are normally key suppressors of effector T cell proliferation [30] . We thus isolated lung CD4 + T cells and analysed their proliferation after in vivo treatment either with recombinant IL-17A or with anti-IL-17A antibody given intranasally. In vivo treatment with recombinant IL-17A (rc IL-17A) in this murine model of lung tumour significantly reduced and conversely, in vivo anti-IL-17A antibody treatment significantly increased, lung CD4 + T cell proliferation ex vivo ( Fig. 5a,b , respectively) in wild-type littermates. Moreover, in contrast to wild-type mice, we found that anti-IL-17A antibody treatment did not further augment proliferation of the already hyper-proliferating lung CD4 + T cells in the T-bet-deficient mice bearing tumours ( Fig. 5c ). 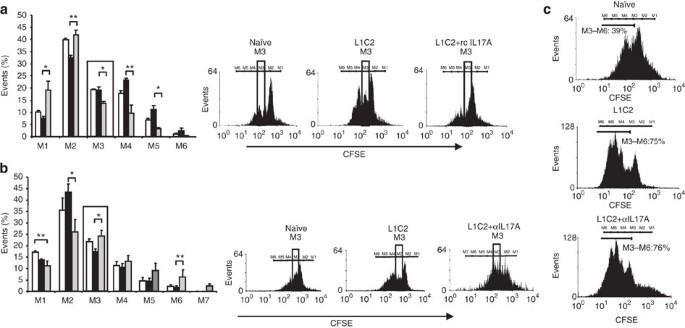Figure 5: Treatment with anti-IL-17A antibodies-induced effector CD4+T cell proliferation. (a) Lung CD4+T cells from naive BALB/cJ wild-type mice (open column) or mice injected with the tumour cell line L1C2 either untreated (black column) or treated with 750 ng rcIL-17A (grey column) on days 5 and 8 after tumour cell injection were isolated on day 21 after tumour cell injection and stained with carboxyfluorescein succinimidyl ester (CFSE). After 4 daysin vitroculture with αCD3/αCD28 antibodies CFSE staining was measured by flow cytometry (N=3–5 per group; representative of 2 independent experiments). (b) Naive lung CD4+T cells (open column) or T cells isolated from wild-type mice bearing L1C2 tumour either untreated (black column) or treated with αIL17A antibody on days 5 and 8 after tumour cell injection (grey column) were isolated 21 days after tumour cell injection and stained with CFSE. At 4 days afterin vitroculture with αCD3/αCD28 antibodies cells were analysed by flow cytometry (N=2–4 per group; representative of 3 independent experiments). (c) T-bet(−/−)CD4+T cells from naive or L1C2-tumour-bearing mice untreated or treated with αIL17A antibody were stained with CFSE. At day 4,in vitroculture with αCD3/αCD28 antibodies CFSE-staining was measured by flow cytometry (three independent experiments). M: Mitosis. Data are shown as mean values±s.e.m. Student's two-tailedt-test was used *P,0.05; **P,0.01. Figure 5: Treatment with anti-IL-17A antibodies-induced effector CD4 + T cell proliferation. ( a ) Lung CD4 + T cells from naive BALB/cJ wild-type mice (open column) or mice injected with the tumour cell line L1C2 either untreated (black column) or treated with 750 ng rcIL-17A (grey column) on days 5 and 8 after tumour cell injection were isolated on day 21 after tumour cell injection and stained with carboxyfluorescein succinimidyl ester (CFSE). After 4 days in vitro culture with αCD3/αCD28 antibodies CFSE staining was measured by flow cytometry ( N =3–5 per group; representative of 2 independent experiments). ( b ) Naive lung CD4 + T cells (open column) or T cells isolated from wild-type mice bearing L1C2 tumour either untreated (black column) or treated with αIL17A antibody on days 5 and 8 after tumour cell injection (grey column) were isolated 21 days after tumour cell injection and stained with CFSE. At 4 days after in vitro culture with αCD3/αCD28 antibodies cells were analysed by flow cytometry ( N =2–4 per group; representative of 3 independent experiments). ( c ) T-bet (−/−) CD4 + T cells from naive or L1C2-tumour-bearing mice untreated or treated with αIL17A antibody were stained with CFSE. At day 4, in vitro culture with αCD3/αCD28 antibodies CFSE-staining was measured by flow cytometry (three independent experiments). M: Mitosis. Data are shown as mean values±s.e.m. Student's two-tailed t -test was used * P ,0.05; ** P ,0.01. Full size image Consistent with the increased immunosuppression in tumours, we detected increased numbers of GITR + CD4 + CD25 + Foxp3 + T regulatory cells in the lungs of tumour-bearing mice. Local treatment with recombinant IL-17A in vivo did not change the number of CD4 + CD25 + Foxp3 + T regulatory cells, whereas conversely anti-IL-17A antibody treatment suppressed the number of these cells in the lungs of wild-type mice as compared with the IgG-treated group ( Fig. 6a ). We then asked whether increasing concentrations of anti-IL-17A antibody would affect tumour growth. Although we did not notice any improvement in the tumour growth by increasing twofold the doses of anti-IL-17A antibodies in vivo , we found a dose-dependent decrease in the number of tumour-associated CD4 + CD25 + Foxp3 + T regulatory cells after anti-IL-17A antibody treatment ( Fig. 6b ). These data suggest that there is already sufficient IL-17A production in vivo such that addition of exogenous IL-17A has no effect, whereas neutralization of IL-17A with anti-IL-17A antibodies has marked effects on regulatory T cells. Moreover, T-bet-deficient mice bearing lung tumours showed an augmented number of CD4 + CD25 + Foxp3 + T regulatory cells and an upregulation of IL-10, an immunosuppressive cytokine, in the supernatants of lung CD4 + T cells compared with wild-type littermates in this tumour model ( Fig. 6c,d , respectively). IL-6, a cytokine known to induce Th 17 cells and suppress Foxp3-expressing cells, was increased in the supernatants of CD4 + T cells isolated from the lung of tumour-bearing T-bet-deficient mice ( Fig. 6e ). Moreover, IL-6 is a cytokine released by CD4 + T cells producing IL-17A. Thus, the increase of IL-6 in the supernatants of lung CD4 + T cells from T-bet-deficient mice supports a role for T-bet on the Th 17 induction in this tumour model mediated by IL-6. Finally, the increased release of IL-17A by lung CD4+ T cells isolated from the lung of T-bet-deficient mice bearing tumours could induce IL-6 production in tumour cells as demonstrated in vitro . To further examine this point, we analysed IL-6 production in tumour-bearing mice and found a significant induction of IL-6 mRNA in the lung of T-bet-deficient mice bearing tumours as compared with the wild-type littermates indicating a role of IL-6 in lung carcinoma in T-bet-deficient mice ( Fig. 6f ). 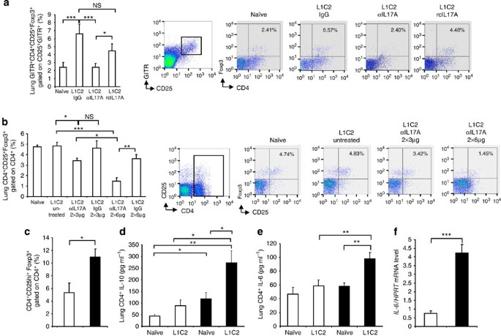Figure 6: IL-17A and T-bet regulate the number of tumour-infiltrating T-regulatory cells. (a) Total lung cells of naive or L1C2-tumour-bearing BALB/cJ wild-type mice untreated or treated on days 5 and 8 with rcIL-17A (2×250 ng) or αIL-17A antibodies (2×3 μg) or control IgG were analysed on day 21 after tumour cell injection by flow cytometry for GITR+CD4+CD25+Foxp3+cells (N=4–5 per group). (b) Flow cytometry analysis of total lung cells of naive or L1C2-tumour-bearing mice untreated or treated with IgG or αIL17A antibodies on days 5 and 8 with either 3 or 6 μg each (N=2–4 per group). (c) Flow cytometric analysis of lung CD4+CD25hi Foxp3+cells of BALB/cJ wt (open columns) and T-bet(−/−)(filled columns) L1C2-tumour-bearing mice (N=2–5 per group; representative of 3 independent experiments). (d,e) Lung CD4+T cells from naive and L1C2-tumour-bearing wild-type (open columns) and T-bet(−/−)(filled columns) mice were isolated and after 24 h cell culture with αCD3/αCD28 antibodies the supernatants were analysed for IL-10 (d) and IL-6 (e) protein levels by ELISA (d:N=3–5 per group, representative of 2 independent experiments;e:N=3–5 per group). (f) qPCR analysis of IL-6 mRNA expression in the lungs of BALB/cJ wt (open columns) and T-bet(−/−)(filled columns) L1C2-tumour-bearing mice (N=5 per group). Data are shown as mean values±s.e.m. Student's two-tailedt-test was used *P,0.05; **P,0.01; ***P,0.001. Figure 6: IL-17A and T-bet regulate the number of tumour-infiltrating T-regulatory cells. ( a ) Total lung cells of naive or L1C2-tumour-bearing BALB/cJ wild-type mice untreated or treated on days 5 and 8 with rcIL-17A (2×250 ng) or αIL-17A antibodies (2×3 μg) or control IgG were analysed on day 21 after tumour cell injection by flow cytometry for GITR + CD4 + CD25 + Foxp3 + cells ( N =4–5 per group). ( b ) Flow cytometry analysis of total lung cells of naive or L1C2-tumour-bearing mice untreated or treated with IgG or αIL17A antibodies on days 5 and 8 with either 3 or 6 μg each ( N =2–4 per group). ( c ) Flow cytometric analysis of lung CD4 + CD25hi Foxp3 + cells of BALB/cJ wt (open columns) and T-bet (−/−) (filled columns) L1C2-tumour-bearing mice ( N =2–5 per group; representative of 3 independent experiments). ( d , e ) Lung CD4 + T cells from naive and L1C2-tumour-bearing wild-type (open columns) and T-bet (−/−) (filled columns) mice were isolated and after 24 h cell culture with αCD3/αCD28 antibodies the supernatants were analysed for IL-10 ( d ) and IL-6 ( e ) protein levels by ELISA ( d : N =3–5 per group, representative of 2 independent experiments; e : N =3–5 per group). ( f ) qPCR analysis of IL-6 mRNA expression in the lungs of BALB/cJ wt (open columns) and T-bet (−/−) (filled columns) L1C2-tumour-bearing mice ( N =5 per group). Data are shown as mean values±s.e.m. Student's two-tailed t -test was used * P ,0.05; ** P ,0.01; *** P ,0.001. Full size image IL-23/IL-23R levels in lung tumour and their dependence on T-bet IL-23 is a tumour-inducing cytokine, released by antigen-presenting cells, involved in the expansion of the Th 17 pathway [31] , [32] , [33] , [34] , [35] , [36] , [37] . We thus looked at IL-23 and IL-23R mRNA levels in the lung. IL-23 levels were significantly higher in T-bet-deficient mice bearing tumours as compared with control wild-type mice ( Fig. 7a ). Furthermore, IL-23R expression was not significantly different between lung CD4 + T cells from wild-type mice and T-bet-deficient mice suggesting that these cells can respond to local IL-23 stimulation ( Fig. 7b ). These findings are consistent with the idea that the absence of T-bet favours a Th17 cytokine response in the lung via IL-23 in experimental lung tumours. 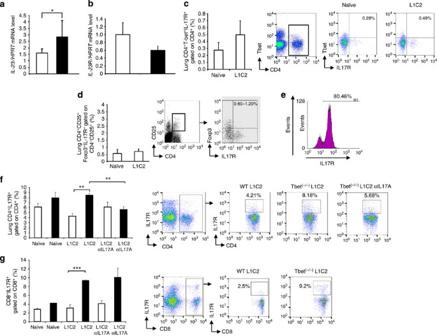Figure 7: T-bet counteracts IL-17A via inhibition of IL-17R signalling on lung CD4+T cells. (a) qPCR analysis of IL-23 expression in wt (open column) and T-bet(−/−)(filled column) total lung cells 21 days after injection of the tumour cell line L1C2 (N=5 per group). (b) IL-23R expression in lung naive CD4+T cells of wt (open column) and T-bet(−/−)(filled column) mice (N=5 per group). (c) Flow cytometric analysis of IL-17R expression on CD4+T-bet+cells of naive and L1C2-tumour-bearing wt mice 21 days after injection of the tumour cells (N=5 mice per group; representative of 3 independent experiments). (d) Flow cytometric analysis of IL-17R on CD4+CD25+Foxp3+T cells of naive and L1C2-tumour-bearing wt mice 21 days after injection of the tumour cells (N=3–5 mice per group; representative of 3 independent experiments). (e) IL-17R expression on L1C2 tumour cells by flow cytometry (representative of three independent experiments). (f,g) Total lung cells isolated from naive and tumour-bearing wt (open columns) and T-bet(−/−)(filled columns) mice untreated or treated with αIL17A antibody on day 5 and 8 were analysed 14 days after tumour cell injection. The number of CD4+IL-17R+cells (f) and CD8+IL-17R+lung cells is shown (N=2–3 per group). Data are shown as mean values±s.e.m. Student's two-tailedt-test was used. *P,0.05; **P,0.01; ***P,0.001. Figure 7: T-bet counteracts IL-17A via inhibition of IL-17R signalling on lung CD4 + T cells. ( a ) qPCR analysis of IL-23 expression in wt (open column) and T-bet (−/−) (filled column) total lung cells 21 days after injection of the tumour cell line L1C2 ( N =5 per group). ( b ) IL-23R expression in lung naive CD4 + T cells of wt (open column) and T-bet (−/−) (filled column) mice ( N =5 per group). ( c ) Flow cytometric analysis of IL-17R expression on CD4 + T-bet + cells of naive and L1C2-tumour-bearing wt mice 21 days after injection of the tumour cells ( N =5 mice per group; representative of 3 independent experiments). ( d ) Flow cytometric analysis of IL-17R on CD4 + CD25 + Foxp3 + T cells of naive and L1C2-tumour-bearing wt mice 21 days after injection of the tumour cells ( N =3–5 mice per group; representative of 3 independent experiments). ( e ) IL-17R expression on L1C2 tumour cells by flow cytometry (representative of three independent experiments). ( f , g ) Total lung cells isolated from naive and tumour-bearing wt (open columns) and T-bet (−/−) (filled columns) mice untreated or treated with αIL17A antibody on day 5 and 8 were analysed 14 days after tumour cell injection. The number of CD4 + IL-17R + cells ( f ) and CD8 + IL-17R + lung cells is shown ( N =2–3 per group). Data are shown as mean values±s.e.m. Student's two-tailed t -test was used. * P ,0.05; ** P ,0.01; *** P ,0.001. Full size image T-bet inhibits IL-17R levels in tumour-infiltrating CD4 + T cells We then hypothesized that the development of Th 1 cells induced by anti-IL-17A antibody treatment might be explained by the presence of an IL-17A-mediated autocrine mechanism on CD4 + T cells. Accordingly, we examined IL-17R expression on lung CD4 + T cells in the presence and absence of the tumour. We found that lung CD4 + T cells do not co-express IL-17R when T-bet or Foxp3 are expressed ( Fig. 7c,d , respectively). However, IL-17R was expressed on the surface of the tumour cell line L1C2 used to induce experimental adenocarcinoma ( Fig. 7e ). Moreover, some CD4 + T cells in the lung expressed the IL-17R and this receptor was upregulated in lung tumour-infiltrating CD4 + and CD8 + T cells of T-bet-deficient mice as compared with wild-type controls ( Fig. 7f,g , respectively). Finally, in vivo anti-IL-17A antibody treatment resulted in reduction of IL-17R expression on the surface of tumour-infiltrating lung CD4 + T cells ( Fig. 7f ) but not in CD8 + T cells in the lungs of T-bet-deficient mice ( Fig. 7g ). Taken together, these data suggest that T-bet suppresses Th 17 responses by inhibiting both IL-17A and IL-17R expression thus interfering with the autocrine and paracrine loops involved in the development of this pathway in CD4 + T cells-infiltrating lung tumours. Here we investigated the role of Th 17 cells in tumours and their relationship with T-bet and Foxp3. We found an upregulation of the Th 17 cell lineage associated with elevated Foxp3 levels in patients with lung adenocarcinoma. Furthermore, we demonstrated that targeting of IL-17A is beneficial in experimental lung cancer by inhibiting lung tumour-infiltrating T regulatory cells and inducing IFN-γ-producing CD4 + T cells in the presence of T-bet. Our findings suggest that IL-17A inhibitors could have broad clinical applications in lung cancer by inhibiting Th 17 and T-regulatory cells in the presence of T-bet. Moreover, in the absence of T-bet, anti-IL-17A antibody therapy could also be partly effective resulting in reduction of IL-17R expression on CD4 + T cells and upregulation of IFN-γ-producing CD8 + T cells with tumour killing function. Although this experimental tumour model does not reflect various characteristics of human lung cancer growth as compared with orthotopic transplantation models with human tissue in immunocompromised mice [38] , [39] , this approach permitted the analysis of antitumour T cell-mediated immune responses in mice with a normal immune system. Using this model we could demonstrate a key role for IL-17A in regulating tumour development in vivo . Our studies in patients with lung adenocarcinoma revealed an inverse correlation between local T-bet and IL-17A levels. In addition, using the experimental lung adenocarcinoma model we uncovered a major role for T-bet in regulating IL-23 and IL-17A levels in the lung. We found that IL-23 levels are significantly higher in lungs from T-bet-deficient mice bearing tumours as compared with wild-type controls suggesting that the tumour environment creates an IL-23-rich milieu favouring Th17 development. Furthermore, although it has been previously demonstrated that silencing of T-bet downregulates IL-23R expression in other experimental settings [40] , we found no difference in IL-23R mRNA levels between lung CD4 + T cells from wild-type and T-bet-deficient mice suggesting that T cells from the latter mice can respond to IL-23 in the lung. In any case, IL-17R-expressing CD4 + T cells were significantly augmented in the lung of T-bet-deficient mice compared with controls indicating a marked regulatory effect of T-bet on lung Th17 cell development. Moreover, we reported here that the tumour cell line used for the in vivo studies produces cytokines favouring Th17 cell development. In particular, this cell line spontaneously released TGF-β and produced IL-6 upon IL-17 stimulation, suggesting that in addition to T-bet levels in T cells, soluble factors produced by the tumour may control the local development of Th17 cells in lung adenocarcinoma. The i.n. administration of low doses of anti-IL-17A antibodies led to a significant suppression of tumour growth as compared with untreated and control IgG-treated mice suggesting a key functional role for IL-17A in controlling tumour growth in vivo . This observation was associated with marked changes in the composition and cytokine production of tumour infiltration T cells. In addition to effector T cells, changes in regulatory T cells were noted in the lung of tumour-bearing mice upon anti-IL-17A treatment. The Th 17 lineage of T lymphocytes has been thought to be in a reciprocal relationship with the development of CD4 + CD25 + Foxp3 + T regulatory cells. In fact, the cytokine IL-6, together with TGF-β 1 has been shown to favour Th 17 development [41] , [42] , whereas it inhibits development of T regulatory cells in vitro and in vivo . CD4 + CD25 + Foxp3 + T regulatory cells are known to suppress the immune responses against tumours, whereas the role of Th 17 cells in lung tumours is not fully understood. Here, we found that the main transcription factors of human Th 17 cells as well as the main transcription factor of T regulatory cells, Foxp3, were increased in lung tumour tissues obtained from patients with lung adenocarcinoma compared with control tissues indicating a dysregulation of these two T cell subsets in lung tumours, resulting in a parallel expansion of both local Th 17 and T reg responses. These findings suggested a potential direct relationship between both T cell lineages in lung cancer. This possibility could also be linked to the differentiation of inducible regulatory T cells [36] . Indeed, we demonstrated that anti-IL-17A antibody treatment decreases the number of lung CD4 + CD25 + Foxp3 + T cells in the presence of T-bet and resulted in amelioration of tumour growth in lung adenocarcinoma. This beneficial effect of anti-IL-17A antibody therapy was accompanied by decreased IL-6 levels and the presence of tumour-infiltrating lung CD4 + T cells that released more IFN-γ and TNFα. These findings suggested that a key target of IL-17A are lung CD4 + T cells, which express the IL-17R and inhibition of this interaction leads to decreased production of IL-6. These results are in agreement and extend the findings in other settings of tumours [25] , [27] . In fact, these authors described a tumour-inducing function of IL-17A and demonstrated that targeted deletion of IL-17A in an IFN-γ-deficient background could ameliorate the tumour load. We further demonstrated that IL-17A is induced in T-bet-deficient mice and might contribute to tumour growth by directly driving IL-6 production by tumour cells. In any case, the reduction of regulatory T cells upon anti-IL-17A antibody treatment is likely to be relevant for the control of tumour growth, as T regulatory cells have been demonstrated to have a pathogenic immunosuppressive role in the tumour [43] , [44] . T-bet has been previously shown to control Th 1 cytokine production in autoimmunity [45] and allergic asthma [46] . Furthermore, T-bet regulates NK cell activity in melanoma [20] , [21] , [47] . The present findings using T-bet knockout mice and in vivo imaging of tumour growth in experimental lung cancer suggest that T-bet is a key regulator of antitumour T cell responses and modulates T reg activity in lung cancer in vivo . We also showed that IL-17A-deficiency leads to increased IFN-γ levels in the airways confirming a reciprocal regulation of Th1 and IL-17A levels in tumours also observed by others [27] . In addition, we found that anti-IL-17A antibody treatment induced IFN-γ expression by CD8 + T cells isolated from the lungs of T-bet-deficient mice as compared with those isolated from wild-type littermates bearing tumours treated the same way. These data correlate with a previously reported distinct effect of T-bet in CD4 + and CD8 + T cells [48] . In conclusion, in experimental lung adenocarcinoma we demonstrated that local blockade of IL-17A leads to suppression of tumour growth and an induction of IFN-γ production by CD4 + T cells, while inhibiting lung CD4 + CD25 + Foxp3 + T regulatory cells in the presence of T-bet. We further found that T-bet inversely correlated with IL-17A levels in patients with lung adenocarcinoma. Furthermore, the anti-IL-17A therapy in the absence of T-bet was partially effective and was associated with decreased IL-17R expression on CD4 + and increased IFN-γ release by lung CD8 + T cells, resulting in an increased survival of T-bet-deficient mice bearing tumours. Such an advantage should be considered for future tailored therapy in the absence of T-bet. Thus, anti-IL-17A antibody therapy emerges as an attractive approach for lung adenocarcinoma. Human subjects and study population Lung specimens were derived from the routine surgical pathology service in an anonymous fashion from the tumour tissue bank of the program project (SFB432) supported by the Deutsche Forschungsgemeinschaft. The study was performed in agreement with the local ethics review board of Rheinland-Pfalz. Quantitative Real-Time PCR in human samples Total cellular RNA was extracted from frozen tissue specimens using RNeasy Mini Kits (Qiagen). The resulting RNA (5 μg) was primed with a dT 18 oligonucleotide and reverse transcribed with Superscript II (Invitrogen) according to the manufacturer's instructions. Integrity of the obtained cDNA was tested by amplification of p53 transcripts in a 30-cycle PCR (sense, 5′-CGTGAGCGCTTCGAGATGTTCCG-3′; antisense, 5′-CCTAACCAGCTGCCCAACTGTAG-3′; annealing temperature 67 °C). The individual gene-specific primer sets were designed to span exon/intron boundaries and quality controlled by PCR reactions using either DNA or not reverse transcribed RNA as template. For PCR analysis of individual gene transcripts, 0.5 μl first-strand cDNA was amplified with transcript-specific oligonucleotides (Operon), using 1 U Hot Star Taq DNA Polymerase (Qiagen) in a 30 μl reaction mixture, according to manufacturer's instructions. The primer sequences and the respective annealing temperatures were as follows: HPRT (sense 5′-TGACACTGGCAAAACAATGCA-3′; antisense 5′-GGTCCTTTTCACCAGCAAGCT-3′; annealing temperature 62 °C), RORα4 (sense 5′-TGTACTGATGTCAGCAGATCG-3′; antisense 5′-ATGAAGTCGCACAATGTCTGG-3′; annealing temperature 60 °C), RORC2 (sense 5′-AAAGCATCCTGGCAAAGCTGC-3′; antisense 5′-TCTTCCAGGTCACTTGGACAG-3′; annealing temperature 60 °C), IL-17A (sense 5′-TCACCTTGGAATCTCCACCGCA-3′; antisense 5′-GGCAGTGTGGAGGCTCCCTG-3′; annealing temperature 60 °C), Foxp3 (sense 5′-CAAGGCTTCATCTGTGGCATC-3′; antisense 5′-CGTGTGAACCAGTGGTAGATC-3′; annealing temperature 60 °C) and T-bet (sense 5′-CCCTTGGTGTGGACTGAGAT-3′; antisense 5′-GTCGGTGTCCTCCAACCTAA-3′; annealing temperature 60 °C). Quantitative RT-PCR analysis was performed using the ABI PRISM 3700 Sequence Detection System instrument and software (Applied Biosystems) with the QuantiTect SYBR Green PCR Kit (Qiagen). Reactions were performed for 40 cycles in triplicates with specific primers (300 nM each) with initial denaturation/activation for 15 min at 95 °C, 30 s denaturation at 95 °C, 30 s annealing, and 30 s amplification at 72 °C. The relative expression level of specific transcripts was calculated with respect to the internal standard, hypoxanthine-guanine-phosphoribosyltransferase (HPRT), to normalize for variances in the quality of RNA and the amount of input cDNA. Expression levels were normalized to normal lung tissues using ΔΔCT calculation. In each experiment, a template-free negative control was included. Cells The L1C2 (Line 1 alveolar cell carcinoma) adenocarcinoma cell line was cultured in RPMI 1640 medium enriched with 10% fetal calf serum (FCS) (Biofluids) and 1% penicillin/streptavidin (Gibco, Invitrogen) antibiotics as previously described [47] . Lewis lung carcinoma cell line (LLC1) was obtained from the American Type Culture Collection (ATCC), and cultured in DMEM with 10% FCS and 1% penicillin/streptavidin. Both cell lines were tested negative for mycoplasma and other transmissible infectious agents. The LL/2-luc-M38 Bioware Cell line (Caliper LifeSciences) was cultured in DMEM with 10% FCS and 1% penicillin/streptavidin. Mice BALB/cJ and C57/BL6 wild-type mice (6–12 weeks old) were maintained under specific pathogen-free conditions. T-bet (−/−) mice were on a Balb/cJ genetic background. These mice were generously given to us by Professor L.H. Glimcher, Harvard Medical School (Boston, MA). IL-17 (−/−) mice were provided by Regeneron Pharmaceuticals on a C57BL/6 background. Wild-type littermates were used as controls. All experiments in mice were done under the licence number 23177-07/G09-1-008 in Mainz and under the licence number IR5520301020 in Erlangen, Germany. Murine model of lung adenocarcinoma and antibody treatment For the adenocarcinoma mouse model a total of 2×10 5 L1C2 cells (in 0.2 ml RPMI medium) were injected into the tail vein of BALB/cJ wt and T-bet (−/−) -mice [49] . In experiments with wt and T-bet-deficient mice, mice were killed on day 14 after tumour cell injection. In experiments using BALB/cJ wt mice only, the animals were killed at day 21. Lungs were removed and analysed as described below. For the treatment with αIL17A antibody and recombinant IL-17A mice received 2×3 or 2×6 μg of anti-IL-17A (goat-anti-mouse antibody, R&D Systems) antibodies or control IgG antibody (goat IgG, R&D Systems) or 2×250 or 2×750 ng recombinant IL-17A (R&D Systems) in 50 μl PBS by i.n. application on days 5 and 8 or days 8 and 11 after intravenous injection of L1C2 cells. For the Lewis lung carcinoma (LLC1) mouse model, 2.2×10 5 LLC1 cells, resuspended in DMEM without supplements, were injected into the tail vein of C57BL/6 wt and IL-17A-deficient mice. At day 21 the animals were killed and analysed. Patho-histological analysis of the lungs For histological analysis, lung samples were immersed in 10% buffered formalin before embedding in paraffin. Tumour load for each lung was quantified by a pathologist (H.-A.L). Three histological step sections were cut at 200 μm intervals from the paraffin block of each lung sample. The slides were stained with haematoxylin and eosin and examined using a diagnostic microscope for the presence of tumour foci. Tumour-containing slides were then photographed using a diagnostic microscope (Olympus BX45) and a digital camera (Olympus C4040) at ×4 magnification and imported as jpg files into Photoshop (Adobe Photoshop, version CS3). Using the pencil tool, the metastases were marked, the surface was covered by a tumour quantified using the histogram (number of pixels/total magnification), and set in relation to the surface covered by the lung (number of pixels/total magnification). Mean values were calculated for each lung based on the analysis of the three sections. In order to avoid observer bias, the morphometric analyses were performed while the pathologist was blinded to the group assignment of the lung samples. Isolation of lung CD4 + and CD8 + T cells Total lung cell suspension and CD4 + /CD8 + T lung cell isolation were performed as previously described [50] . Isolated T cells were cultured with plate-bound anti-CD3 antibody (CD3 clone 145-2C11, 5 μg ml −1 ) and soluble anti-CD28 antibody (CD28 clone 37.51, 2 μg ml −1 , BD Biosciences-PharMingen) for 20 h at a density of 10 6 cells ml −1 . Supernatants were collected, frozen and subsequently analysed for cytokine production by enzyme-linked immunosorbent assay (ELISA). FACS analysis and surface marker staining Total lung cells (5×10 5 ) were washed with 1 ml PBS and incubated with 5 μg ml −1 of different FACS antibodies for 30 min at 4 °C. Afterwards the cells were washed with 1 ml PBS and measured by FACS Calibur and analysed by using Cell Quest Pro version 4.02 (BD Biosciences) or by Flow-Jo 7.6 (Tree Star). The following anti-mouse FACS antibodies were used: CD4 PE or CD4 PerCP (BD Biosciences RM4-5), CD8a APC (BD Biosciences 53-6.7), IL-17R-FITC or IL-17R-PE (R&D Systems), CD25 PE (eBioscience PC61.5), and GITR-FITC (eBioscience DTA-1). To assure the purity of CD4 + T cell isolation, anti-mouse CD4-APC antibody (L3T4 BD Biosciences) was used. Intracellular staining Freshly isolated total lung cells (1.5×10 6 ) were washed with 1 ml PBS, and incubated for 30 min at 4 °C with the surface FACS antibodies. After washing cells were fixed and permeabilized with Fixation/Permeabilization concentrate/diluent (eBioscience) and stained in 10× Permeabilization Buffer (eBioscience) for the intracellular proteins according to the manufacturer's protocol. The following intracellular anti-mouse antibodies were used: Foxp3-APC (eBioscience FJK-16s) and T-bet-Alexa fluor 647 (eBioscience). In-vitro analysis of lung CD4 + cells CD4 + T cells were isolated from naive and tumour-bearing lungs 6 days after intravenous injection of 2×10 5 L1C2 cells. Lung CD4 + T cells were then re-stimulated in-vitro with anti-CD3 antibody (5 μg ml −1 ), anti-CD28 antibody (2 μg ml −1 ), IL-2 (25 U ml −1 ) and with either anti-IL-17A antibody (5 μg ml −1 ) or IgG control for 3 days in culture. Afterwards IFN-γ was measured in the cell supernatant by ELISA. ELISA All cytokines in the supernatants were detected by specific sandwich ELISA sets. TNFα, IFN-γ, IL-10 and IL-6 ELISA sets (BD Biosciences), and IL-17A and TGFβ ELISA sets (R&D Systems) were used according to the manufacturer's protocol. Luciferase measurement The luciferase-expressing LL/2-luc-M38 Bioware cell line (1 million cells per mouse per 200 μl) was injected in the tail vein of C57BL/6 mice. At different time points the mice were injected intraperitonally with 150 μl luciferin (15 mg ml −1 ), anaesthetised with isoflurane and luciferase activity was measured with the Caliper Ivis System by detecting the luminescence intensity to determine the tumour load in the lungs. The analysis was done in a logarithmic scale mode. For tumour load quantification the total flux (photons per second) was determined. Tumour cell in vitro culture The tumour cells (62.500 cells per ml) were cultured for 48 h with different concentrations of recombinant IL-17A (0–500 ng ml −1 ) and αIL-17A antibody (1 μg ml −1 ) (R&D systems). TGF-β levels in the supernatants were measured by ELISA as described above. Total RNA of the tumour cells was extracted and after cDNA synthesis (Fermentas) gene expression of the tumour cells was determined by qPCR (quantitative real-time PCR) using the following primers: IL-6 fwd. : 5′-AGTTGCCTTCTTGGGACTGA-3′; IL-6 rev. : 5′-TCCACGATTTCCCAGAGAAC-3′. Statistical analysis Differences were evaluated for significance ( P <0.05) by the Student's two-tailed t -test for independent events (Excel, PC). Where indicated statistical comparison was performed by using analysis of the variance. Data are given as mean values±s.e.m. How to cite this article: Reppert, S. et al . A role for T-bet-mediated tumour immune surveillance in anti-IL-17A treatment of lung cancer. Nat. Commun. 2:600 doi: 10.1038/ncomms1609 (2011).